Quantum Hall effect on top and bottom surface states of topological insulator (Bi1−xSbx)2Te3films The three-dimensional topological insulator is a novel state of matter characterized by two-dimensional metallic Dirac states on its surface. To verify the topological nature of the surface states, Bi-based chalcogenides such as Bi 2 Se 3 , Bi 2 Te 3 , Sb 2 Te 3 and their combined/mixed compounds have been intensively studied. Here, we report the realization of the quantum Hall effect on the surface Dirac states in (Bi 1− x Sb x ) 2 Te 3 films. With electrostatic gate-tuning of the Fermi level in the bulk band gap under magnetic fields, the quantum Hall states with filling factor ±1 are resolved. Furthermore, the appearance of a quantum Hall plateau at filling factor zero reflects a pseudo-spin Hall insulator state when the Fermi level is tuned in between the energy levels of the non-degenerate top and bottom surface Dirac points. The observation of the quantum Hall effect in three-dimensional topological insulator films may pave a way toward topological insulator-based electronics. Quantum transport in Dirac electron systems has been attracting much attention for the half-integer quantum Hall effect (QHE), as typically observed in graphene [1] , [2] . A single Dirac fermion under a magnetic field is known to show the quantized Hall effect with the Hall conductance σ xy =( n +1/2) e 2 / h with n being an integer, e the elemental charge and h the Planck constant. This 1/2 is the characteristic of the Dirac fermion compared with the usual massive electrons. In graphene with such a Dirac electron, however, there is fourfold degeneracy due to the spin and valley degrees of freedom, and hence the quantized Hall conductance shows up experimentally as σ xy =4( n +1/2) e 2 / h . The recently discovered topological insulator (TI) possesses metallic Dirac states on the edge or surface of an insulating bulk [3] , [4] , [5] , [6] . With the application of a magnetic field ( B ), the unique features of Dirac bands may be exemplified via the formation of Landau levels (LLs). The QHE is the hallmark of dissipationless topological quantum transport originating from one-dimensional chiral edge modes driven by cyclotron motion of two-dimensional (2D) electrons. Unlike the case of graphene, the degeneracy is completely lifted in the spin-polarized Dirac state of 2D and three-dimensional (3D) TIs. The Hall conductance σ xy of 3D TI is expected to be given by the sum of the two contributions from the top and bottom surfaces and hence σ xy =( n + n ’+1) e 2 / h with both n and n ’ being integers. When the two contributions are equivalent, that is, n = n ’, only the odd integer QHE is expected. For such 3D TI films, the top and bottom surfaces support surface states with opposite spin-momentum locked modes when the top and bottom surfaces are regarded as two independent systems. Such a helicity degree of freedom in real space can be viewed as the pseudo-spin variable and is hence expected to yield a new quantum state via tuning of surface magnetism and/or Fermi level ( E F ) that is applicable to quantum computation functions [7] , [8] , [9] . Although intensive research has been carried out for bulk crystals, thin films and field-effect devices [10] , [11] , [12] , [13] , [14] , [15] , [16] , [17] , parasitic bulk conduction and/or disorder in the devices continues to hamper efforts to resolve quantum transport characteristics of the Dirac states on chalcogenide 3D TIs surfaces. The most venerable example of the QHE with least bulk conduction has been achieved in a 70 nm strained HgTe film [18] . Compared with the HgTe system, 3D-TIs of Bi-chalcogenides such as Bi 2 Se 2 Te and (Bi 1− x Sb x ) 2 Te 3 have a good potential for exploring the Dirac surface states with wide controllability of transport parameters (resistivity, carrier type and density) and band parameters (energy gap, position of Dirac point and Fermi velocity) by changing the compositions [19] , [20] . In the following, we report on the QHE in field-effect transistors based on 3D TI thin films of (Bi 1− x Sb x ) 2 Te 3 ( x =0.84 and 0.88). With electrostatic gate-tuning of the Fermi level in the bulk band gap under magnetic fields, quantized Hall plateaus ( σ xy =± e 2 / h ) at the filling factor ν =±1 are resolved, pointing to the formation of chiral edge modes at the top/bottom surface Dirac states. In addition, the emergence of a σ xy =0 state around the charge neutral point (CNP) reflects a pseudo-spin Hall insulator state when the location of Fermi level is between the non-degenerate top and bottom surface Dirac points. Transport properties with electrostatic gate-tuning We grew 3D TI thin films of (Bi 1− x Sb x ) 2 Te 3 ( x =0.84 and 0.88; both 8 nm thick) using molecular beam epitaxy (MBE) [19] and insulating InP (111) substrates. The E F of as-grown film was tuned near to the bulk band edge by precisely controlling the Bi/Sb composition ratio [19] , [20] . Films were then fabricated into photolithography-defined gated Hall-bar devices to allow electrostatic tuning of E F . A cross-sectional schematic of the device structure and the top-view image are shown in Fig. 1a,b , respectively. The device consists of a Hall bar defined by Ar ion-milling, and an atomic-layer-deposited AlO x insulator isolated Ti/Au top gate with electron-beam-evaporated Ti/Au electrodes (see Methods). The magnetotransport measurements were carried out in a dilution refrigerator by low-frequency (3 Hz) lock-in technique with a low excitation current of 1 nA to suppress heating (see Supplementary Fig. 1 and Supplementary Note 1 ). 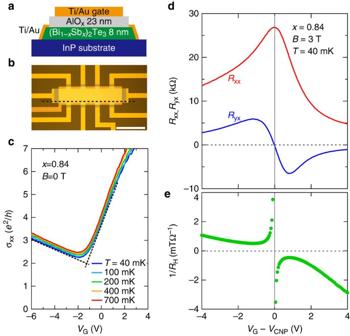Figure 1: Gating of topological insulator (Bi0.16Sb0.84)2Te3thin film. (a,b) Cross-sectional schematic and top-view photograph of a Hall-bar device. Broken line inbindicates the position fora. Scale bar, 300 μm. (c) Top gate voltageVGdependence of longitudinal conductivityσxxat various temperatures. (d,e) Effective gate voltage (VG−VCNP) dependence of longitudinal and transverse resistance (RxxandRyx) and inverse of Hall coefficient 1/RHunder magnetic fieldB=3 T at temperatureT=40 mK. TheVGfor the charge neutral point (CNP),VCNP, is defined as the gate voltage whereRyxis crossing zero. Figure 1: Gating of topological insulator (Bi 0.16 Sb 0.84 ) 2 Te 3 thin film. ( a , b ) Cross-sectional schematic and top-view photograph of a Hall-bar device. Broken line in b indicates the position for a . Scale bar, 300 μm. ( c ) Top gate voltage V G dependence of longitudinal conductivity σ xx at various temperatures. ( d , e ) Effective gate voltage ( V G − V CNP ) dependence of longitudinal and transverse resistance ( R xx and R yx ) and inverse of Hall coefficient 1/ R H under magnetic field B =3 T at temperature T =40 mK. The V G for the charge neutral point (CNP), V CNP , is defined as the gate voltage where R yx is crossing zero. Full size image First, device operation was examined at B =0 T. Figure 1c shows the electric field effect controlled conductivity σ xx of the x =0.84 film as a function of top gate voltage V G with changing temperature. The minimum conductivity of roughly 2 e 2 / h is observed at V G =−1.7 V. On both sides of this minimum, σ xx shows a linear but asymmetric increase with increasing or decreasing V G . The weak temperature dependence of longitudinal conductivity σ xx for a wide range of V G is characteristic of the gapless nature of Dirac states under finite disorder [21] . Thus, we ascribe the conductivity of this TI film below 1 K to the Dirac surface states with a small contribution from bulk conduction. To verify the ambipolar nature of the device, the longitudinal and transverse resistance R xx and R yx as a function of V G at B =3 T were measured ( Fig. 1d ). As expected, this results in a sign change of R yx at a certain V G , which we hereafter define as the gate voltage corresponding to E F being located at the charge neutral point (CNP), V CNP. This point coincides closely with the V G at which R xx reaches a maximum. At the V CNP , the Hall effects from the top and bottom surface states appear to cancel, resulting in R yx ∼ 0, although electron-rich and hole-rich puddles are thought to still exist, as in the case of graphene [22] . To capture the essence of the observed phenomena, we hereafter take the working hypothesis that E F shifts equally on top and bottom states, which in turn retain their difference in energy position. The inverse of Hall coefficient 1/ R H is shown in Fig. 1e , which would be proportional to 2D charge carrier density n 2D =1/( eR H ), in the simplest case. Asymmetric behaviour of 1/ R H between positive and negative V G regions with respect to V CNP is in accord with the asymmetric σ xx behaviour at zero magnetic field as shown in Fig. 1c . The more efficient increase in σ xx with electron accumulation (positive V G ) is often observed in ambipolar TI transistors [13] , [14] , [15] , [16] , [17] and may be related to the difference in v F (Fermi velocity) above and below the Dirac point [19] . In addition, the proximity of the Dirac point to the valence band edge needs to be taken into account for the present thin film system; in most of the negative region of V G − V CNP , E F must go inside the valence band in which doped holes appears to be fully localized at low temperatures below 1 K, as argued later. Observation of quantum Hall states With applying higher magnetic field of B =14 T, clear signatures of QHE are revealed in the temperature dependence of R xx and R yx , as shown in Fig. 2a–d for the x =0.84 film and in Fig. 2e–h for the x =0.88 film. We first focus on the results of the x =0.84 film. R xx increases steeply with lowering the temperature for V G corresponding to the CNP, yet decreases rapidly toward zero on both sides at higher and lower V G . Concomitantly to the decrease in R xx , R yx reaches the values of quantum resistance ± h / e 2 =±25.8 kΩ and forms plateaus in V G at T =40 mK. This correspondence between the rapidly declining R xx value and the quantized R yx plateaus at ± h / e 2 are distinct evidence for QHE at Landau filling factor ν =±1, respectively, as schematically shown in Fig. 2i (magnetic field dependence is shown in Supplementary Fig. 2 and discussed in Supplementary Note 2 ). The LL splitting energy of Dirac dispersion ( E n ) is given by , where n is the LL index. 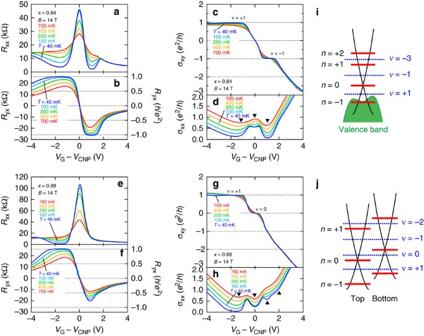Figure 2: Observation of the quantum Hall effect. (a,b,e,f), Effective gate voltageVG−VCNPdependence ofRxxandRyxat various temperatures ofT=40–700 mK with application of magnetic fieldB=14 T for thex=0.84 (a,b) andx=0.88 (e,f) films of (Bi1−xSbx)2Te3. (c–e,h), Effective gate voltageVG−VCNPdependence ofσxxandσxyat various temperatures ofT=40–700 mK with the application of magnetic fieldB=14 T for thex=0.84 andx=0.88 films of (Bi1−xSbx)2Te3as deduced from the correspondingRxxandRyxdata. Triangles indandhshow the dips ofσxx. (i) Schematics of the Landau levels (LLs) of the surface state of (Bi1−xSbx)2Te3(x=0.8–0.9) thin film in case of the degenerate top and bottom surface state. At a high field, for example, 14 T, then=−1 LL of the surface state locates below the top of the valence band. When the Fermi energy (EF) is tuned between the LLs, the quantum Hall state with indexνemerges. (j) Schematics of the LLs of the top and bottom surface states in case then=0 (Dirac point) energy is different between the two surfaces. Figure 2: Observation of the quantum Hall effect. ( a , b , e , f ), Effective gate voltage V G − V CNP dependence of R xx and R yx at various temperatures of T =40–700 mK with application of magnetic field B =14 T for the x =0.84 ( a , b ) and x =0.88 ( e , f ) films of (Bi 1− x Sb x ) 2 Te 3 . ( c – e , h ), Effective gate voltage V G − V CNP dependence of σ xx and σ xy at various temperatures of T =40–700 mK with the application of magnetic field B =14 T for the x =0.84 and x =0.88 films of (Bi 1− x Sb x ) 2 Te 3 as deduced from the corresponding R xx and R yx data. Triangles in d and h show the dips of σ xx . ( i ) Schematics of the Landau levels (LLs) of the surface state of (Bi 1− x Sb x ) 2 Te 3 ( x =0.8–0.9) thin film in case of the degenerate top and bottom surface state. At a high field, for example, 14 T, the n =−1 LL of the surface state locates below the top of the valence band. When the Fermi energy ( E F ) is tuned between the LLs, the quantum Hall state with index ν emerges. ( j ) Schematics of the LLs of the top and bottom surface states in case the n =0 (Dirac point) energy is different between the two surfaces. Full size image Using the data of R xx and R yx , σ xy and σ xx as functions of V G − V CNP for the x =0.84 film are plotted in Fig. 2c,d . Again, the Hall plateaus at σ xy =± e 2 / h as well as minima of σ xx approaching zero (black triangles) are observed and are indicative of the QHE with ν =±1. In this plot, however, two additional features are to be noted. The first is an unexpectedly wide σ xy plateau and thermally activated behaviour of σ xx for the ν =+1 ( σ xy = e 2 / h ) state in the corresponding V G − V CNP (negative) region. As already noted in the V G asymmetric change of σ xx ( Fig. 1c ) in the negative region of V G − V CNP , that is, hole-doping, E F readily reaches the valence band top. The energy position of Dirac point of the x =0.84 film lies by at most 30 meV above the valence band top, while the LL splitting between n =0 and n =−1 levels amounts to 70 meV at 14 T, according to resonant tunneling spectroscopy on similarly grown thin films of (Bi 1− x Sb x ) 2 Te 3 (ref. 19 ). From the consideration of the Fermi velocity of Dirac cone, the V G − V CNP value at which the E F reaches the valence band top is estimated to be around −1.5 V or even a smaller absolute value. Therefore, in the V G − V CNP region where the quantum Hall plateau or its precursor is observed, the E F locating between n =0 and n =−1 LLs of the surface state is close to or already buried in the valence band, as schematically shown in Fig. 2i . Although the doped but localized holes in the valence band may hardly contribute to transport, that is, σ xy (bulk) ≪ σ xy (surface), the relative E F shift with negatively sweeping V G − V CNP becomes much slower as compared with the positive sweep case owing to the dominant density of states of the valence band. This explains a wider plateau region for ν =+1 in the hole-doping side, contrary to the normal behaviour of electron accumulation side, ν =−1. The second notable feature in Fig. 2c is the emergence of the ν =0 state around V G = V CNP , as seen in the step of σ xy and (finite) minimum in σ xx as functions of V G − V CNP . This state is more clearly resolved in the x =0.88 film, as shown in Fig. 2e–h , on which we focus hereafter. In a similar manner to the x =0.84 film, the x =0.88 film also shows with lowering temperature divergent behaviour of R xx around V G = V CNP , while approaching zero around V G − V CNP =−1.5 V. The similar divergent (at V G = V CNP ) and vanishing (at V G − V CNP =−1.5 V) behaviours of R xx are observed also with increasing B at 40 mK (see Supplementary Fig. 3 and Supplementary Note 3). The R yx reaches 25.8 kΩ around V G − V CNP =−1.5 V forming the ν =+1 quantum Hall state, whereas in the electron-doping regime, R yx reaches −20 kΩ, short of the quantized value. The failure to form the fully quantized ν =−1 state is perhaps related to the disorder of the surface Dirac state, which is induced by the compositional/structural disorder of the as-grown film and cannot be overcome by gate tuning. Nevertheless, the ν =0 feature is clearly resolved for the x =0.88 film, as shown in the V G dependence of σ xy ( Fig. 2g ) calculated from R xx and R yx . In addition to the σ xy = e 2 / h ( ν =+1) plateau, a plateau at σ xy =0 appears at around V G = V CNP . The plateau broadening occurs via centring at σ xy =0.5 e 2 / h as the isosbestic point with elevating temperature. In accordance with the plateaus in σ xy , σ xx takes a minima at ν =+1 and 0, as shown in Fig. 2h . Here, we can consider the contribution of both the top and bottom surface Dirac states to this quantization of σ xy , as schematically shown in Fig. 2j . At the ν =+1 ( ν =−1) state, both the top and bottom surfaces are accumulated by holes (electrons) with E F being located between n =0 and n =−1 ( n =+1) LLs, giving rise to the chiral edge channel. In contrast, we assign the ν =0 state to the gapping of the chiral edge channel as the cancellation of the contributions to σ xy from the top and bottom surface states with ν =±1/2, when E F locates in between the energy levels of the top and bottom surface Dirac points ( n =0 levels), as shown in Fig. 2j . This ν =0 state can hence be viewed as a pseudo-spin Hall insulator, if we consider the top and bottom degree of freedom as the pseudo-spin variable. Such an observation of a zero conductance plateau has been reported also in disordered graphene under very high magnetic field [23] , [24] , [25] , [26] and analysed theoretically [27] , as well as in the 2D TIs, the quantum wells of HgTe [28] and InAs/GaSb [29] . From the analyses shown in the following, we propose here that the major origin for the presence of σ xy =0 is more like the energy difference of the top/bottom Dirac points rather than other effects such as electron-hole puddles due to composition inhomogeneity. To further discuss the characteristics of these QH states, we investigate the B dependence of σ xy ( Fig. 3a,b ). 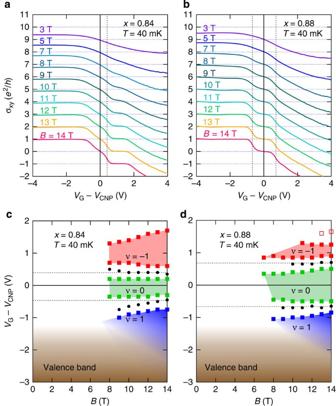Figure 3: Magnetic field dependence of Hall plateaus. (a,b)σxyatT=40 mK under variousBas a function of effective gate voltageVG−VCNPfor thex=0.84 (a) andx=0.88 (b) films. Traces for lower magnetic fields are each vertically offset bye2/h. Dotted lines represent the plateau transitions as defined atσxy=±0.5e2/h. (c,d) Quantizedσxyphase diagram for theν=+1, 0 and −1 (blue, green and red shaded, respectively) states associated with the plateau edges (filled squares) and the plateau transition point (filled circles) defined atσxy=±0.5e2/hin the plane of magnetic field andVG−VCNP. The plateau edges are determined by the second-orderVGderivative ofσxy. The analysis of the plateau width against V G determines the phase diagram as shown in Fig 3c,d . The plateau edges are determined from the second derivative of σ xy with respective to V G (see Supplementary Fig. 4 and Supplementary Note 4), while the plateau transition points between ν =0 and ν =±1 are defined here by σ xy =± e 2 /2 h . The plateau shrinks with decreasing B for the ν =−1 state of the x =0.84 film ( Fig. 3a ). However, the ν =+1 state for both films appears to be rather robust with reducing V G (doping more holes), since E F positions already below the top of the valence band, perhaps for V G − V CNP <−1.5 V. On the other hand, the ν =0 plateau is only weakly dependent on B , although the plateau width is wider for x =0.88 than for x =0.84. The observation of ν =0 requires the condition that the Fermi level is located in between the energy levels of the top and bottom surface Dirac points ( Fig. 2j ). From the Hall data in the relatively high positive V G − V CNP region (electron-doping) shown in Fig. 1e , we can know the relation between the sum of the top and bottom Dirac electron density versus V G − V CNP . Then, with the values of the ν =0 plateau width between the σ xy =±0.5 e 2 / h points ( δV G ∼ 0.9 and 1.4 V; see Fig. 3c,d ) and the Fermi velocity ( v F ∼ 5 × 10 5 ms −1 ; ref. 19 ), we can estimate the energy difference ( δE DP ) between the Dirac points at the top and bottom surface states to be ∼ 50 meV and ∼ 70 meV for the x =0.84 and x =0.88 film, respectively (see Supplementary Note 5 ). These values should be compared with a much larger band gap energy ( ∼ 250 meV). The energy difference δE DP is, however, considerably larger than a Zeeman shift ( ∼ 9 meV at 14 T; ref. 19 ), which rationalizes the above analysis with ignoring the Zeeman shift of the n =0 LL. Although the reason why the two films ( x =0.84 and 0.88) show such a difference in δE DP is not clear at the moment, we speculate that the monolayer buffer layer of Sb 2 Te 3 ( x =1.0) used for the growth of the x =0.88 film (see Methods) may cause the considerably higher energy position of the Dirac point at the bottom surface. Incidentally, for the region of | V G − V CNP |< δV G /2, electron accumulation at the top surface and hole accumulation at the bottom surface should coexist. This may naturally explain the observed ( Fig. 1e and see also Supplementary Fig. 5 and Supplementary Note 6) deviation from the linear relationship between 1/ R H and V G − V CNP as well as the extrema of 1/ R H observed at around ± δV G /2. Figure 3: Magnetic field dependence of Hall plateaus. ( a , b ) σ xy at T =40 mK under various B as a function of effective gate voltage V G − V CNP for the x =0.84 ( a ) and x =0.88 ( b ) films. Traces for lower magnetic fields are each vertically offset by e 2 / h . Dotted lines represent the plateau transitions as defined at σ xy =±0.5 e 2 / h . ( c , d ) Quantized σ xy phase diagram for the ν =+1, 0 and −1 (blue, green and red shaded, respectively) states associated with the plateau edges (filled squares) and the plateau transition point (filled circles) defined at σ xy =±0.5 e 2 / h in the plane of magnetic field and V G − V CNP . The plateau edges are determined by the second-order V G derivative of σ xy . 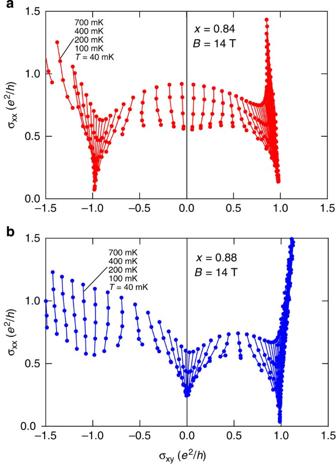Figure 4: Flows ofσxyandσxx. (a,b) (σxy,σxx) are displayed with the two experimental subparameters (TandVG) for the x=0.84 (a) and x=0.88 (b) films. Each line connecting between points represents the flow behaviour of (σxy,σxx) with lowering temperature from 700 to 40 mK at the specific value ofVGatB=14 T. The flows direct from upper to lower with decreasing temperature. Full size image Figure 4 summarizes the flow of conductivity tensor ( σ xy , σ xx ) plotted with the two experimental subparameters ( T and V G ) at 14 T. With decreasing T , the flow in ( σ xy , σ xx ) tends to converge toward either of ( σ xy , σ xx )=(− e 2 / h , 0), (0, 0) or ( e 2 / h , 0) at high magnetic field (for example, 14 T), which corresponds to ν =−1, 0 and +1 QH state, respectively. Incipient convergence to ν =0 is discerned for the x =0.84 film ( Fig. 4a ), while the ν =−1 state is not discernible for the x =0.88 film ( Fig. 4b ). Among these three QH states, the unstable fixed point appears to lie on the line of σ xy =±0.5 e 2 / h (approximately with the critical σ xx value of ∼ 0.5 e 2 / h ) which corresponds to the crossing of E F at the n =0 LL (or Dirac point) of the bottom and top surface state (see Fig. 2j ), respectively [30] . Figure 4: Flows of σ xy and σ xx . ( a , b ) ( σ xy , σ xx ) are displayed with the two experimental subparameters ( T and V G ) for the x=0.84 ( a ) and x=0.88 ( b ) films. Each line connecting between points represents the flow behaviour of ( σ xy , σ xx ) with lowering temperature from 700 to 40 mK at the specific value of V G at B =14 T. The flows direct from upper to lower with decreasing temperature. Full size image In conclusion, we have successfully observed the QHE at ν =±1 and 0 in 3D TI thin films of (Bi 1− x Sb x ) 2 Te 3 ( x =0.84 and 0.88). Due to a considerable difference of the Dirac point (or n =0 LL) energies of the top and bottom surfaces of the thin film, the ν =0 state observed at σ xy =0 is interpreted as a pseudo-spin Hall insulator with the top/bottom degree of freedom as the pseudo-spin. Further studies on non-local transport in mesoscopic structures will open the door to dissipationless topological-edge electronics on the basis of the 3D topological insulators. MBE film growth Thin films of (Bi 1− x Sb x ) 2 Te 3 ( x =0.84 and 0.88) were fabricated by MBE on semi-insulating InP (111) substrate. The Bi/Sb composition ratio was calibrated by the beam equivalent pressure of Bi and Sb, namely 8 × 10 −7 Pa and 4.2 × 10 −6 Pa for x =0.84 and 6 × 10 −7 Pa and 4.4 × 10 −6 Pa for x =0.88. The Te flux was over-supplied with the Te/(Bi+Sb) ratio kept at ∼ 20. The substrate temperature was 200 °C and the growth rate was ∼ 0.2 nm per minute. Fabrication procedures for the x =0.84 and 0.88 films are slightly different at the initial growth on InP surfaces. We grew the 0.84 film with supplying Te and (Bi+Sb) from the initial stage. For the x =0.88 film, we started with supplying Te and Sb for a monolayer growth of Sb 2 Te 3 buffer layer followed by Bi shutter opening. This difference may be an origin of the larger energy gap δE DP of the Dirac points between the top and bottom surfaces ( Fig. 2j ) for the x =0.88 film. After the epitaxial growth of 8 nm-thick thin films, in situ annealing was performed at 380 °C to improve surface morphology. Device fabrication The AlO x capping layer was deposited at room temperature with an atomic layer-deposition system immediately after the discharge of the samples from MBE. This process turned out to be effective to protect the surface from degradation. The device structure was defined by subsequent photolithography and Ar ion-milling processes. Ohmic-contact electrodes and top gate electrode were Ti/Au and deposited with an e-beam evaporator. Here, ion-milling was performed under 45-degree tilt condition on a rotating stage, resulting in the ramped side edge as schematically shown in Fig. 1a . This ensured electrical contact to the top and bottom of the film. How to cite this article: Yoshimi, R. et al , Quantum Hall effect on top and bottom surface states of topological insulator (Bi 1− x Sb x ) 2 Te 3 films. Nat. Commun , 6:6627 doi: 10.1038/ncomms7627 (2015).